NF-Y inactivation causes atypical neurodegeneration characterized by ubiquitin and p62 accumulation and endoplasmic reticulum disorganization Nuclear transcription factor-Y (NF-Y), a key regulator of cell-cycle progression, often loses its activity during differentiation into nonproliferative cells. In contrast, NF-Y is still active in mature, differentiated neurons, although its neuronal significance remains obscure. Here we show that conditional deletion of the subunit NF-YA in postmitotic mouse neurons induces progressive neurodegeneration with distinctive ubiquitin/p62 pathology; these proteins are not incorporated into filamentous inclusion but co-accumulated with insoluble membrane proteins broadly on endoplasmic reticulum (ER). The degeneration also accompanies drastic ER disorganization, that is, an aberrant increase in ribosome-free ER in the perinuclear region, without inducing ER stress response. We further perform chromatin immunoprecipitation and identify several NF-Y physiological targets including Grp94 potentially involved in ER disorganization. We propose that NF-Y is involved in a unique regulation mechanism of ER organization in mature neurons and its disruption causes previously undescribed novel neuropathology accompanying abnormal ubiquitin/p62 accumulation. Nuclear transcription factor-Y (NF-Y), also known as the CCAAT binding factor, is an evolutionarily conserved transcription factor composed of three subunits; NF-YA, NF-YB and NF-YC. It binds to CCAAT motif in the proximal promoter region to induce gene expression [1] . NF-Y has been shown to regulate an increasing number of genes because of its general binding consensus and its ubiquitous expression. This suggests multiple roles of NF-Y in various contexts. Previously, Bhattacharya et al. [2] have shown that NF-YA knockout in mice leads to early embryonic lethality, and its knockout in embryonic fibroblasts suppresses cell-cycle progression and then induces apoptosis. The involvement of NF-Y in cell-cycle regulation and apoptosis has also been reported in several tumour cell lines [3] , [4] , [5] . Furthermore, recent observations highlight the role of NF-Y in stem cell progression and maintenance. For example, in skeletal muscle cells, NF-Y is active for proliferation in myoblasts, and then becomes inactive during differentiation due to downregulation of NF-YA [6] , [7] , [8] . A similar pattern of NF-Y involvement has been reported in hematopoietic stem cells [9] , [10] , and in this case its in vivo significance has been confirmed in NF-YA knockout mice [11] . Finally, NF-Y appears to be required for embryonic stem cell proliferation, whereas expressions of some of NF-Y subunits are downregulated during differentiation [12] . Thus, one of the essential functions of NF-Y is the cell-cycle regulation in proliferating cells, which is important for cell proliferation and maintenance, and possibly also for tumour progression and embryogenesis. Although NF-Y activity is often declined during differentiation as described above, we have recently found that NF-Y is expressed and still active in mature neurons of adult mouse brain [13] . In addition, NF-Y is suppressed by mutant huntingtin containing expanded polyglutamine during disease progression in Huntington’s disease (HD) model [13] . NF-Y suppression has also been reported in other neurodegenerative diseases caused by polyglutamine expansion, such as spinal and bulbar muscular atrophy and spinocellebular ataxia 17 (refs 14 , 15 ). Thus, at least in neurons, NF-Y is active even after differentiation and its suppression may be involved in some aspects of neurodegeneration. However, the actual neuronal function of NF-Y remains to be clarified. In this study, we find that conditional deletion of NF-YA in mouse brain postmitotic neurons induces progressive neurodegeneration. Notably, the degeneration accompanies distinctive ubiquitin (Ub)/p62 pathology, that is, Ub and p62 are not incorporated into filamentous inclusion but co-accumulated with insoluble membrane proteins broadly on endoplasmic reticulum (ER). The NF-YA deletion also induces an aberrant increase in smooth ER (SER) in the perinuclear region without causing an unfolded protein response (UPR), a major adaptive response to ER stress. We further perform chromatin immunoprecipitation–DNA microarray (ChIP–chip) and identify several NF-Y target genes possibly involved in ER disorganization. These data indicate that NF-Y is involved in a novel regulation mechanism of ER organization independently of UPR in mature neurons and its disruption results in neuronal loss with atypical neurodegenerative features including abnormal Ub/p62 accumulation and drastic SER increase. Neuronal NF-YA deletion causes progressive neurodegeneration To inactivate NF-Y in differentiated neurons, we used NF-YA flox mice in which exons 3–8 out of 9 total coding exons are flanked by loxP sequences ( Fig. 1a ) [2] . For conditional deletion, we used camk2a-cre transgenic mice that express cre specifically in forebrain differentiated neurons [16] . By using RNZ reporter mice that express LacZ in nuclei through cre-mediated recombination [17] , [18] , we confirmed specific recombination by the camk2a-cre transgene in the forebrain region, especially in the cortex and hippocampus ( Fig. 1d ) [19] . Through several rounds of crossing, we obtained two NF-YA conditional deletion mice: NF-YA flox/flox; cre and flox/−; cre mice (see Methods for detail). 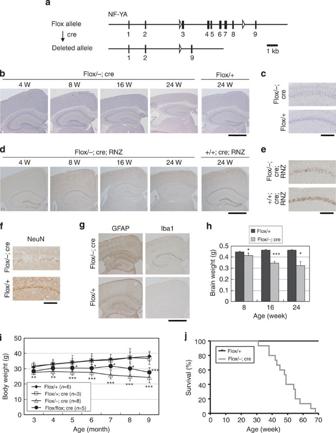Figure 1: Conditional deletion ofNF-YAin neurons induces progressive neurodegeneration and shortens lifespan. (a) Gene structure ofNF-YAflox and deleted allele. Two inserted flox sequences are indicated as triangles. Exons 3–8 are deleted by cre-mediated gene recombination. (b) Hematoxylin staining of coronal sections ofNF-YAflox/−; cre and flox/+ mice at indicated weeks of age. (c) Hematoxylin-stained hippocampal CA1 region of 16-week-old mice. (d) Anti-LacZ staining of coronal sections ofRNZreporter mice harbouringNF-YAflox/−; cre or +/+; cre at indicated weeks of age. (e) Anti-LacZ-stained CA1 regions of 8-week-old mice. (f) CA1 regions of anti-NeuN-stained coronal sections of 8-week-old mice. (g) Anti-GFAP and Iba1 staining of coronal sections of 8-week-old mice. (h) Brain weights of mice of indicated weeks of age. Values are means±s.d. of at least three mice (*P<0.05, ***P<0.001,t-test). (i) Body weights of mice harbouring indicated genotypes (n means number of analysed mice). Values are means±s.d. (*P<0.05, **P<0.01, ***P<0.001,t-test). (j) Survival rates ofNF-YAflox/−; cre (n=15) and flox/+ (n=12) mice. The median survival of flox/−; cre mice is 47.5 weeks (P<0.0001, log-rank test). Scale bars are 1 mm (b,d,g) and 200 μm (c,e,f). Figure 1: Conditional deletion of NF-YA in neurons induces progressive neurodegeneration and shortens lifespan. ( a ) Gene structure of NF-YA flox and deleted allele. Two inserted flox sequences are indicated as triangles. Exons 3–8 are deleted by cre-mediated gene recombination. ( b ) Hematoxylin staining of coronal sections of NF-YA flox/−; cre and flox/+ mice at indicated weeks of age. ( c ) Hematoxylin-stained hippocampal CA1 region of 16-week-old mice. ( d ) Anti-LacZ staining of coronal sections of RNZ reporter mice harbouring NF-YA flox/−; cre or +/+; cre at indicated weeks of age. ( e ) Anti-LacZ-stained CA1 regions of 8-week-old mice. ( f ) CA1 regions of anti-NeuN-stained coronal sections of 8-week-old mice. ( g ) Anti-GFAP and Iba1 staining of coronal sections of 8-week-old mice. ( h ) Brain weights of mice of indicated weeks of age. Values are means±s.d. of at least three mice (* P <0.05, *** P <0.001, t -test). ( i ) Body weights of mice harbouring indicated genotypes (n means number of analysed mice). Values are means±s.d. (* P <0.05, ** P <0.01, *** P <0.001, t -test). ( j ) Survival rates of NF-YA flox/−; cre ( n =15) and flox/+ ( n =12) mice. The median survival of flox/−; cre mice is 47.5 weeks ( P <0.0001, log-rank test). Scale bars are 1 mm ( b , d , g ) and 200 μm ( c , e , f ). Full size image We then examined brain structure by staining sections with Hematoxylin. We found that the cortex and hippocampus of NF-YA deletion mice were structurally unaffected at 4 weeks but then became degenerated during ageing ( Fig. 1b,c ). Analysis of mice at later stage with different genotypes confirmed that the degeneration is specific to the NF-YA deletion mice ( Supplementary Fig. 1 ). Progressive reduction of LacZ staining in RNZ mice indicated loss of NF-YA deletion neurons during ageing ( Fig. 1d,e , Supplementary Table 1 ). Indeed, the cells positive for the neuronal marker NeuN were reduced compared with the control ( Fig. 1f ). In contrast, GFAP-positive astrocytes and Iba1-positive microglia were increased ( Fig. 1g ). Finally, the mice showed progressive reduction in brain weight ( Fig. 1h , Supplementary Fig. 2a ). These data clearly indicate that conditional deletion of NF-YA induces progressive neurodegeneration accompanying gliosis. The NF-YA deletion mice also showed progressive reduction of body weight and shortened life spans ( Fig. 1i,j , Supplementary Fig. 2b–d ). Thus, the neurodegeneration results in body weight loss. Neuronal NF-Y inactivation induces Ub and p62 accumulation Accumulation of Ub and a scaffold protein p62/Sqstm1 with fibrillar protein aggregates is a well-known neuropathology often observed in various neurodegenerative diseases [20] , [21] . We examined its involvement in the NF-YA deletion-induced degeneration and found that Ub and p62 were progressively accumulated in the cortex and hippocampus of NF-YA deletion mice ( Fig. 2a,b ). Confocal analysis showed cytoplasmic accumulations of these proteins, and in the case of p62, punctate stainings were also observed ( Fig. 2c , Supplementary Fig. 3 ). Ub was found in NeuN-positive neurons but not in GFAP- or Iba1-positive glia ( Fig. 2d ). However, the cells positive for NeuN staining gradually decreased in the Ub-accumulating cells from 4 weeks (92.3%, n =52), 8 weeks (54.7%, n =150) to 16 weeks (14.0%, n =164) ( n means number of analysed cells) ( Fig. 2d ). Thus, NF-YA deletion induces cytoplasmic accumulations of Ub and p62 in neurons, followed by neuronal loss. 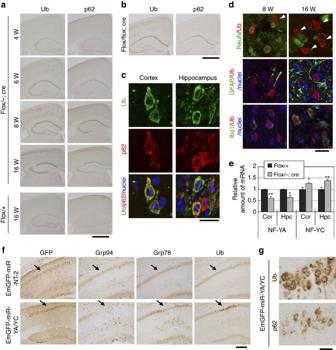Figure 2: Accumulation of Ub and p62 in neurons byNF-YAconditional deletion or NF-YA/NF-YC knockdown. (a) Anti-Ub and p62 staining of coronal sections ofNF-YAflox/−; cre and flox/+ mice at indicated weeks of age. (b) Anti-Ub and p62 staining of coronal section of 8-week-oldNF-YAflox/flox; cre mouse. (c) Confocal analysis of cortical and hippocampal CA1 neurons co-stained with Ub and p62 in 8-week-oldNF-YAflox/−; cre mouse. Nuclei were stained with TOTO-3. (d) Confocal analysis of cortical region co-stained with Ub (red) and NeuN, GFAP or Iba1 (green) inNF-YAflox/−; cre mice at 8 and 16 weeks of age. Nuclei were stained with TOTO-3. Arrowheads indicate Ub-positive cells without NeuN staining, which were increased at 16 weeks of age. (e) Quantitative RT–PCR analysis of NF-YA and NF-YC in cortex (Cor) and hippocampus (Hpc) of 5-week-oldNF-YAflox/−; cre (n=3) or flox/+ (n=3) female mice. Ratios to flox/+ were shown. Values are means±s.d. (*P<0.05, **P<0.01,t-test). (f,g) AAV encoding EmGFP fusing miR-YA/YC (tandem miRNAs against NF-YA and NF-YC) or NT-2 (non-targeting miRNA control) was injected into hippocampal CA1 region of wild-type B6 mice. Mice were fixed at 4 weeks after injection and sections were stained with antibody against GFP, Grp94, Grp78, Ub or p62. (f) Low magnified images. EmGFP-positive CA1 cells are indicated by arrows. (g) High-magnification images of cytoplasmic accumulations of Ub and p62 by miR-YA/YC. Scale bars are 1 mm (a,b), 0.2 mm (f) and 20 μm (c,d,g). Figure 2: Accumulation of Ub and p62 in neurons by NF-YA conditional deletion or NF-YA/NF-YC knockdown. ( a ) Anti-Ub and p62 staining of coronal sections of NF-YA flox/−; cre and flox/+ mice at indicated weeks of age. ( b ) Anti-Ub and p62 staining of coronal section of 8-week-old NF-YA flox/flox; cre mouse. ( c ) Confocal analysis of cortical and hippocampal CA1 neurons co-stained with Ub and p62 in 8-week-old NF-YA flox/−; cre mouse. Nuclei were stained with TOTO-3. ( d ) Confocal analysis of cortical region co-stained with Ub (red) and NeuN, GFAP or Iba1 (green) in NF-YA flox/−; cre mice at 8 and 16 weeks of age. Nuclei were stained with TOTO-3. Arrowheads indicate Ub-positive cells without NeuN staining, which were increased at 16 weeks of age. ( e ) Quantitative RT–PCR analysis of NF-YA and NF-YC in cortex (Cor) and hippocampus (Hpc) of 5-week-old NF-YA flox/−; cre ( n =3) or flox/+ ( n =3) female mice. Ratios to flox/+ were shown. Values are means±s.d. (* P <0.05, ** P <0.01, t -test). ( f , g ) AAV encoding EmGFP fusing miR-YA/YC (tandem miRNAs against NF-YA and NF-YC) or NT-2 (non-targeting miRNA control) was injected into hippocampal CA1 region of wild-type B6 mice. Mice were fixed at 4 weeks after injection and sections were stained with antibody against GFP, Grp94, Grp78, Ub or p62. ( f ) Low magnified images. EmGFP-positive CA1 cells are indicated by arrows. ( g ) High-magnification images of cytoplasmic accumulations of Ub and p62 by miR-YA/YC. Scale bars are 1 mm ( a , b ), 0.2 mm ( f ) and 20 μm ( c , d , g ). Full size image To examine that the observed effects by NF-YA deletion are really caused by suppression of NF-Y, we checked the reduction of NF-YA expression by performing quantitative reverse transcription (RT)–PCR using brain tissue from 5-week-old NF-YA deletion mice in which no significant reduction of brain weight was observed ( Supplementary Fig. 2a ). Using a primer set for exons 7–8 ( Supplementary Fig. 4a ), we found a ~40% reduction in NF-YA mRNA in NF-YA deletion mouse brain ( Fig. 2e ). The reduction of NF-YA protein was confirmed by western blot and immunofluorescence analysis ( Supplementary Fig. 5 ). We also found slight increase in NF-YC ( Fig. 2e , Supplementary Fig .5a,b ), possibly due to its compensatory induction by NF-Y suppression [13] . These data support the notion of NF-YA reduction and NF-Y suppression by NF-YA gene deletion. Unexpectedly, RT–PCR using different primer sets suggested that mutant NF-YA mRNA lacking exons 3–8 region was produced from its deleted allele at high levels ( Supplementary Fig. 4a,b ). To rule out the possibility that this mutant NF-YA itself had some effects, we examined NF-YA heterozygous deletion mice ( NF-YA +/−). Although induction of mutant NF-YA mRNA and partial reduction of full-length mRNA were observed in the brain ( Supplementary Fig. 4c ), these mice showed no reductions in body or brain weights and no inductions of Ub accumulation or gliosis, even in aged mice ( Supplementary Fig. 4d,e ). This suggests that mutant NF-YA mRNA transcribed from its deleted allele has no effect on neurodegeneration. Finally, we found that adeno-associated virus (AAV) vector-mediated knockdown of both NF-YA and NF-YC induced cytoplasmic accumulations of Ub and p62 in hippocampal CA1 cells ( Fig. 2f,g ). Taken together, we conclude that suppression of NF-Y either by gene deletion or by gene knockdown results in Ub and p62 accumulations in brain neurons. Accumulation of membrane proteins with Ub and p62 around ER To examine the mechanism of Ub and p62 accumulations, we performed fractionation analysis using cortical lysates. As shown in Fig. 3a , Ub and p62 were highly detected in the detergent-insoluble fraction from NF-YA deletion mice. In contrast, no clear accumulation was observed for known disease-associated aggregate-prone proteins such as Tau, α-synuclein, FUS/TLS and TDP-43 ( Supplementary Fig. 6a ), suggesting that insolubilization of Ub and p62 is not simply due to aggregation of these proteins. To identify the proteins co-accumulating with Ub and p62, the insoluble fractions were subjected to SDS-PAGE ( Supplementary Fig. 6b ), and then analysed by mass spectrometry. We further checked mRNA levels of the identified proteins to exclude the nonspecifically incorporated proteins such as glial GFAP due to induced gene expression ( Supplementary Fig. 6c ). Finally, around 100 proteins including Ub and p62 were identified to be specifically insolubilized in the cortex of NF-YA deletion mice ( Supplementary Table 2 ). Notably, known aggregate-prone proteins were not identified here, again supporting the idea of no involvement of previously described protein aggregation in the Ub/p62 insolubilization. 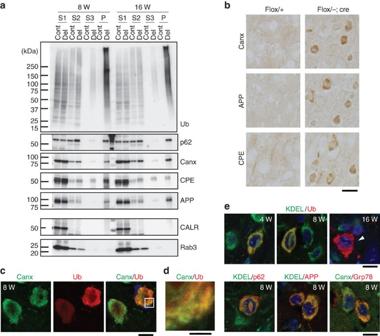Figure 3: Insolubilization and ER accumulation of Ub and p62 and integral membrane proteins inNF-YAdeletion mice. (a) Isolated brain cortexes from 8- or 16-week-oldNF-YAflox/−; cre (Del) and flox/+ (Cont) mice were sequentially solubilized with RIPA (S1), 1% salkosyl/RIPA (S2), 4% salkosyl/RIPA (S3) and formic acid (P) and then analysed by western blotting. Full-size blots can be found inSupplementary Fig. 15. (b) Cortical layer II–III region of 8-week-old mice stained with indicated antibodies. (c) Confocal analysis of cortex of 8-week-oldNF-YAflox/−; cre mice co-stained with antibodies for Canx and Ub. (d) Magnified image of boxed region in (c). (e) Confocal analysis of cortex ofNF-YAflox/−; cre mice co-stained with antibodies as indicated. Nuclei were stained with TOTO-3. Arrowhead indicates Ub-positive cell without KDEL staining. Scale bars are 20 μm (b), 10 μm (c,e) and 5 μm (d). Figure 3: Insolubilization and ER accumulation of Ub and p62 and integral membrane proteins in NF-YA deletion mice. ( a ) Isolated brain cortexes from 8- or 16-week-old NF-YA flox/−; cre (Del) and flox/+ (Cont) mice were sequentially solubilized with RIPA (S1), 1% salkosyl/RIPA (S2), 4% salkosyl/RIPA (S3) and formic acid (P) and then analysed by western blotting. Full-size blots can be found in Supplementary Fig. 15 . ( b ) Cortical layer II–III region of 8-week-old mice stained with indicated antibodies. ( c ) Confocal analysis of cortex of 8-week-old NF-YA flox/−; cre mice co-stained with antibodies for Canx and Ub. ( d ) Magnified image of boxed region in ( c ). ( e ) Confocal analysis of cortex of NF-YA flox/−; cre mice co-stained with antibodies as indicated. Nuclei were stained with TOTO-3. Arrowhead indicates Ub-positive cell without KDEL staining. Scale bars are 20 μm ( b ), 10 μm ( c , e ) and 5 μm ( d ). Full size image We then performed gene ontology (GO) analysis by GO:TermFinder [22] and revealed a significant enrichment of proteins located in membranous cellular compartments including the plasma membrane (45/106, P =3.80E–09), Golgi (29/106, P =7.67E–14), ER (24/106, P =3.53E–08) and cytoplasmic vesicle (20/106, P =9.49E–08). Western blot analysis confirmed the preferential insolubilization of an ER-resident membrane protein, Calnexin, as well as the plasma membrane proteins carboxypeptidase E (CPE) and amyloid beta precursor protein (APP) ( Fig. 3a ). In contrast, an ER luminal protein, calreticulin, and certain cytoplasmic proteins including Rabs (Rab3, 6 and 11), enolase 1 and Arf1, all of which were also found by mass spectrometry ( Supplementary Table 2 ), were not obvious in the insoluble fractions ( Fig. 3a , Supplementary Fig. 6d ). These data suggest the preferential insolubilization of integral membrane proteins together with Ub and p62 in the brains of NF-YA deletion mice. Categorization based on the ontologies suggested insolubilization of membrane proteins with wide cellular distributions from ER to plasma membrane ( Table 1 ). Table 1 List of the insolubilized integral membrane proteins and their intracellular locations. Full size table We next examined the cellular distribution of these insolubilized membrane proteins and found that, similar to Ub and p62, they accumulated in the cytoplasm of cortical neurons in NF-YA deletion mice ( Fig. 3b ). Confocal analysis revealed clear co-distribution of Ub with Calnexin in the cytoplasm ( Fig. 3c,d ), suggesting their accumulation around ER. Indeed, Ub, p62, APP and Calnexin showed clear co-distribution with the ER luminal marker, KDEL (or Grp78) ( Fig. 3e ). However, the cells positive for KDEL staining gradually decreased in the Ub-accumulating cells from 4 weeks (84.5%, n =84), 8 weeks (62.4%, n =101) to 16 weeks (21.0%, n =281) ( n is the number of analysed cells) ( Fig. 3e ), which is almost compatible with the decrease in NeuN staining described above. Taken together, these data indicate that NF-YA deletion induces abnormal accumulation of several membrane proteins, including ER-resident and plasma membrane proteins, around the ER together with Ub and p62, after which ER luminal proteins disappear possibly due to cell degeneration. We also co-stained Ub with the following organelle markers: HSP60, a mitochondrial marker that did not show clear co-distribution with Ub, and GM130, a Golgi marker that was detected in Ub-negative cells but lost in its positive cells ( Supplementary Fig. 7a,b ). Collectively, these data indicate that ER is the organelle that accumulates insolubilized proteins, which may accompany Golgi disassembly. Aberrant increase in SER at perinuclear region We next examined ER morphological alteration by electron microscopy (EM). Analysis of the hippocampal CA1 regions in the NF-YA deletion mice identified cells occupied with reticularly arranged cisternal structures in the large portions of perikarya, in addition to dying cells showing cell shrinkage with an increased electron density ( Fig. 4a,b , Supplementary Fig. 8 ). Nuclear indentations were also observed in these cells ( Fig. 4b ). Detailed analysis clearly showed that these structures resemble ribosome-free SER where the luminal spaces were smaller in width and denser in the electron density than those of control mice ( Fig. 4c,d ). These morphological features, including drastic increase in SER as well as nuclear indentations were also observed in cortical layer II–III neurons of NF-YA deletion mice ( Fig. 4e–g , Supplementary Fig. 8 ). In addition, cytoplasmic components such as free ribosomes (mostly detected as polysomes) were unevenly distributed, that is, abundant in the perinuclear region but sparse in the cell periphery ( Fig. 4f , Supplementary Fig. 8e ), possibly due to suppression of their diffusion in the cytoplasm by increased SER. We further performed immuno-EM and found that Ub and p62 were clearly localized on the membrane of reticularly arranged SER-like structures ( Fig. 4h,i ). Taken together, these data indicate that neuronal deletion of NF-YA induces abnormal increases in SER in the perinuclear region where insolubilized proteins accumulate. 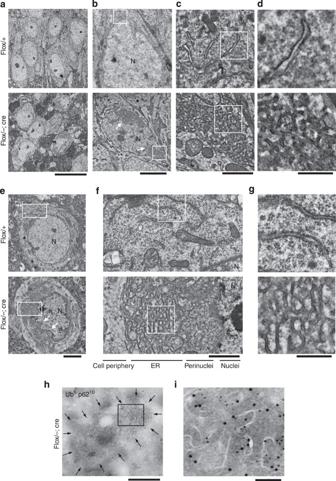Figure 4: Accumulation of reticularly arranged SER-like cisternal structures inNF-YAdeletion mice neurons. (a–d) Electron micrographs of hippocampal CA1 neurons of 8-week-oldNF-YAflox/−; cre or flox/+ mice. (a) Low-magnification images. (b–d) Images with different magnification. Boxed areas are enlarged in the next panels. (e–g) Electron micrographs of cortical layer II–III neurons of 8-week-oldNF-YAflox/−; cre or flox/+ mice. Images with different magnifications are shown. Boxed areas are enlarged in the next panels. Nuclear indentations (arrows inb,e) and nuclear regions (N) are indicated. Subcellular regions are also indicated in case of cortical neurons ofNF-YAdeletion mice (f; lower panel). (h) Double immunogold labelling of Ub (5 nm particles) and p62 (10 nm particles) in a hippocampal CA1 neuron of an 8-week-oldNF-YAflox/−; cre mouse. Immunosignals for Ub and p62 are localized on reticularly arranged membranes of ER-like structures surrounded by arrows. (i) High magnification of boxed region in (h). Scale bars are 20 μm (a), 5 μm (b,e), 1 μm (c,f), 0.2 μm (d,g), 0.5 μm (h) and 0.1 μm (i). Figure 4: Accumulation of reticularly arranged SER-like cisternal structures in NF-YA deletion mice neurons. ( a – d ) Electron micrographs of hippocampal CA1 neurons of 8-week-old NF-YA flox/−; cre or flox/+ mice. ( a ) Low-magnification images. ( b – d ) Images with different magnification. Boxed areas are enlarged in the next panels. ( e – g ) Electron micrographs of cortical layer II–III neurons of 8-week-old NF-YA flox/−; cre or flox/+ mice. Images with different magnifications are shown. Boxed areas are enlarged in the next panels. Nuclear indentations (arrows in b , e ) and nuclear regions (N) are indicated. Subcellular regions are also indicated in case of cortical neurons of NF-YA deletion mice ( f ; lower panel). ( h ) Double immunogold labelling of Ub (5 nm particles) and p62 (10 nm particles) in a hippocampal CA1 neuron of an 8-week-old NF-YA flox/−; cre mouse. Immunosignals for Ub and p62 are localized on reticularly arranged membranes of ER-like structures surrounded by arrows. ( i ) High magnification of boxed region in ( h ). Scale bars are 20 μm ( a ), 5 μm ( b , e ), 1 μm ( c , f ), 0.2 μm ( d , g ), 0.5 μm ( h ) and 0.1 μm ( i ). Full size image Identification of NF-Y-binding gene promoters by ChIP–chip To identify molecular mechanism involved in NF-YA deletion-induced ER pathologies, we tried to identify physiological targets of NF-Y in brain by performing ChIP from wild-type cortex. Three different NF-Y antibodies were used for ChIP of NF-Y, and rabbit IgG and two antibodies for USF1, an E-box interacting transcription factor, were used for control ChIPs. ChIP–PCR confirmed binding of NF-Y and USF1 to known binding promoters, Hspa1a/Dnajb1 and FMR1, respectively ( Fig. 5a ). The NF-Y and rabbit IgG ChIP samples were then subjected to mouse promoter array (chip) and the obtained data were analysed using CisGenome software [23] to identify genomic regions significantly enriched in NF-Y ChIP–chip (the NF-Y ChIP–chip regions) compared with that of rabbit IgG. Analysis of the identified regions showed enrichment of a motif containing the NF-Y-binding consensus, CCAAT ( Fig. 5b ), which is detected in ChIP–chip regions of three NF-Y antibodies ( Fig. 5c ). Gene annotation of these ChIP–chip regions revealed significant overlap among the genes of three NF-Y ChIP samples ( Fig. 5d ). We then picked up the top 400 gene-annotated regions identified in at least two of the NF-Y ChIP–chip data sets ( Supplementary Data 1 ). Detailed analysis revealed an abundance of NF-Y-binding regions around transcription start site (TSS) especially at −500 to 0 bp ( Fig. 5e ). GO analysis by GO:TermFinder [22] showed that, in addition to genes related to transcription (91/423 (21.5%), P =5.98E–09) and cell cycle (40/423 (9.5%), P =2.38E–02), genes involved in stress response (37/423 (8.7%), P =2.41E–03), protein folding (13/423 (3.1%), P =4.20E–03) and protein transport (39/423 (9.2%), P =4.51E–03) were significantly enriched in the 423 identified genes. Among them, we picked up two major ER chaperones, Grp94 and Grp78, because NF-Y binding to their promoters has been reported in different contexts [24] , [25] , and confirmed that NF-Y-binding regions were highly compatible with the positions of the NF-Y-binding consensus ( Fig. 5f,g ). Thus, all of the data indicated that the ChIP–chip worked well and that the obtained genes may be direct targets of NF-Y in the brain. We rechecked the GO of these identified genes, and focused on genes involved in ER function, cytoplasmic protein folding (chaperone) and ubiquitin proteasome system, or vesicle transport. ChIP–PCR confirmed the preferential binding of NF-Y to their promoters ( Fig. 5h , Supplementary Fig. 9 ), which were often higher than those of Hspa1a and Dnajb1, which were not identified by NF-Y–ChIP–chip. Thus, NF-Y could be involved in the regulation of these identified genes, possibly more efficiently than the cytoplasmic chaperones. 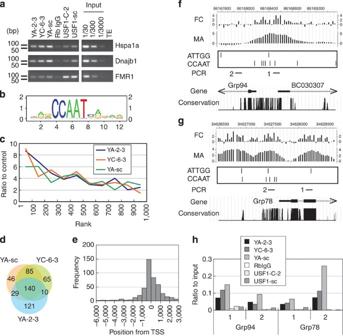Figure 5: Searching NF-Y-binding promoters in mouse brain cortex by ChIP–chip. Cortical lysates from 8-week-old wild-type mice were subjected to ChIP using anti-NF-YA (2-3 or SantaCruz (sc)), anti-NF-YC (6-3), anti-USF1 (C-2 or sc) or control rabbit IgG. The NF-Y and rabbit IgG ChIP samples were subjected to mouse promoter array analysis and NF-Y ChIP–chip regions were obtained. (a) ChIP–PCR for known target gene promoters. Full-size gels can be found inSupplementary Fig. 14. (b) Prediction of NF-Y-binding motif by analysing YA-2-3 ChIP–chip regions. (c) The NF-Y ChIP–chip regions were ranked based on the fold changes, and the frequencies of the NF-Y-binding motif shown in (b) in each 100 regions were analysed. Ratios to matched control genomic regions were plotted. (d) The ChIP–chip regions were gene-annotated and overlapping of top 300 genes was examined among the samples indicated. (e) Top 400 gene promoter regions identified in at least two NF-Y ChIP–chip data sets were picked up, and distances of each ChIP–chip region from a 5′ TSS was analysed. (f,g) The YA-2-3 ChIP–chip regions found in the promoters of Grp94 (f) and Grp78 (g). Fold changes (FC) and moving averages (MA) of neighbouring±five-FCs are shown. Positions of potential NF-Y-binding sites, CCAAT and ATTGG, as well as gene location and conservation are also described. (h) Quantitative ChIP–PCR using two primer sets targeting indicated regions described in (f) and (g). Figure 5: Searching NF-Y-binding promoters in mouse brain cortex by ChIP–chip. Cortical lysates from 8-week-old wild-type mice were subjected to ChIP using anti-NF-YA (2-3 or SantaCruz (sc)), anti-NF-YC (6-3), anti-USF1 (C-2 or sc) or control rabbit IgG. The NF-Y and rabbit IgG ChIP samples were subjected to mouse promoter array analysis and NF-Y ChIP–chip regions were obtained. ( a ) ChIP–PCR for known target gene promoters. Full-size gels can be found in Supplementary Fig. 14 . ( b ) Prediction of NF-Y-binding motif by analysing YA-2-3 ChIP–chip regions. ( c ) The NF-Y ChIP–chip regions were ranked based on the fold changes, and the frequencies of the NF-Y-binding motif shown in ( b ) in each 100 regions were analysed. Ratios to matched control genomic regions were plotted. ( d ) The ChIP–chip regions were gene-annotated and overlapping of top 300 genes was examined among the samples indicated. ( e ) Top 400 gene promoter regions identified in at least two NF-Y ChIP–chip data sets were picked up, and distances of each ChIP–chip region from a 5′ TSS was analysed. ( f , g ) The YA-2-3 ChIP–chip regions found in the promoters of Grp94 ( f ) and Grp78 ( g ). Fold changes (FC) and moving averages (MA) of neighbouring±five-FCs are shown. Positions of potential NF-Y-binding sites, CCAAT and ATTGG, as well as gene location and conservation are also described. ( h ) Quantitative ChIP–PCR using two primer sets targeting indicated regions described in ( f ) and ( g ). Full size image Specific downregulation of Grp94 without modulating UPR To examine the effect of NF-Y suppression on its target gene expressions, we first performed gene expression array using brains from 5-week-old NF-YA deletion mice in which reduction of full-length NF-YA mRNA was observed ( Fig. 2e ). However, not many downregulated genes were obtained (<50 genes showing FC less than −1.2, P <0.05), possibly due to progressive neurodegeneration and high gliosis induction, which makes it difficult to identify altered gene expression in intact neurons. Indeed, expressions of Grp94 and Grp78 were observed in activated microglia ( Supplementary Fig. 7c ). Thus, we used cultured neuro2a cells in which both NF-YA and NF-YC were knocked down ( Supplementary Fig. 10a,b ). Gene expression array revealed reduced expression of some of the genes identified by ChIP–chip in these cells ( Supplementary Fig. 10c ). After validation by quantitative RT–PCR, the following genes were found to be significantly reduced: Grp94, Kdelc1 Rab5b and Tpcn1, whereas moderate reductions were found for Cnpy3, Sdf2l1, Hrd1, Yif1a and Dnajb5 ( Fig. 6a , Supplementary Fig. 10d–f ). Interestingly, no reduced expression was observed for Grp78 and other ER chaperones such as Calnexin and Erdj3, suggesting that NF-Y dependency is different among these ER chaperons in neuro2a cells. 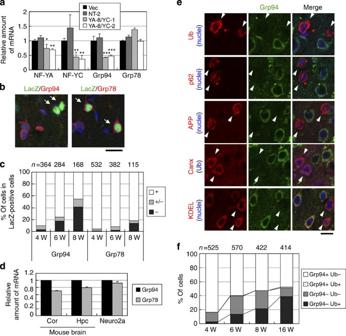Figure 6: Specific reduction of Grp94 expression by NF-Y suppression in neuro2a cells and cortical neurons. (a) Neuro2a cells were transfected with pcDNA6.2-EmGFP vector encoding tandem miRNAs for NF-YA and NF-YC (YA-8/YC-1 or YA-8/YC-2), control miRNA (NT-2) or empty vector (Vec). After 2 days, the cells were subjected to quantitative RT–PCR. Values are means±s.d. of three experiments (*P<0.05, **P<0.01, ***P<0.001,t-test). (b,c) Coronal sections ofRNZreporter mice harbouringNF-YAflox/−; cre were stained with anti-LacZ together with antibodies for Grp94 or Grp78. (b) Confocal images for cortical region of 8-week-old mice. LacZ-positive cells are indicated by arrows. (c) LacZ-positive cells in cortex region were first picked up and then categorized into three groups based on the staining of Grp94 or Grp78; no signal (−), background level (±) or similar to control level (+). Ratios to total LacZ-positive cells are shown (nmeans number of analysed cells). (d) Comparison of endogenous Grp78 mRNA levels with those of Grp94 in mouse brain (8-week-old flox/+ female cortex (Cor) and hippocampus (Hpc)) and neuro2a cells by quantitative RT–PCR using plasmid DNAs containing their cDNAs as standards. Values are means±s.d. of three experiments. (e,f) Coronal sections ofNF-YAflox/−; cre mice were stained with Grp94 (green) together with antibody for Ub, p62, APP, Calnexin or KDEL (red). Nuclei were stained with TOTO-3. (e) Confocal images for cortical region of 8-week-old mice co-stained with antibodies as indicated. Grp94-negative cells are indicated by arrowheads. (f) Cells in cortical region were first categorized into two groups; cells positive (+) or negative (−) for Grp94, and then, staining of Ub in each group of cells was analyzed (nmeans number of analysed cells). Scale bars are 20 μm (b) and 10 μm (e). Figure 6: Specific reduction of Grp94 expression by NF-Y suppression in neuro2a cells and cortical neurons. ( a ) Neuro2a cells were transfected with pcDNA6.2-EmGFP vector encoding tandem miRNAs for NF-YA and NF-YC (YA-8/YC-1 or YA-8/YC-2), control miRNA (NT-2) or empty vector (Vec). After 2 days, the cells were subjected to quantitative RT–PCR. Values are means±s.d. of three experiments (* P <0.05, ** P <0.01, *** P <0.001, t -test). ( b , c ) Coronal sections of RNZ reporter mice harbouring NF-YA flox/−; cre were stained with anti-LacZ together with antibodies for Grp94 or Grp78. ( b ) Confocal images for cortical region of 8-week-old mice. LacZ-positive cells are indicated by arrows. ( c ) LacZ-positive cells in cortex region were first picked up and then categorized into three groups based on the staining of Grp94 or Grp78; no signal (−), background level (±) or similar to control level (+). Ratios to total LacZ-positive cells are shown ( n means number of analysed cells). ( d ) Comparison of endogenous Grp78 mRNA levels with those of Grp94 in mouse brain (8-week-old flox/+ female cortex (Cor) and hippocampus (Hpc)) and neuro2a cells by quantitative RT–PCR using plasmid DNAs containing their cDNAs as standards. Values are means±s.d. of three experiments. ( e , f ) Coronal sections of NF-YA flox/−; cre mice were stained with Grp94 (green) together with antibody for Ub, p62, APP, Calnexin or KDEL (red). Nuclei were stained with TOTO-3. ( e ) Confocal images for cortical region of 8-week-old mice co-stained with antibodies as indicated. Grp94-negative cells are indicated by arrowheads. ( f ) Cells in cortical region were first categorized into two groups; cells positive (+) or negative (−) for Grp94, and then, staining of Ub in each group of cells was analyzed ( n means number of analysed cells). Scale bars are 20 μm ( b ) and 10 μm ( e ). Full size image We then focused on the differential regulation of Grp78 and Grp94 expressions by NF-Y, and examined their in vivo expressions by using the RNZ mice, which expressed LacZ by cre-mediated gene recombination as described above. We found preferential loss of Grp94 but not Grp78 in LacZ-positive cortical cells of NF-YA deletion mice ( Fig. 6b ), which were gradually increased during ageing ( Fig. 6c ). The preferential reduction of Grp94 was further confirmed by AAV-mediated knockdown of NF-YA and NF-YC in hippocampal CA1 neurons ( Fig. 2f ). Quantitative analysis using plasmid DNAs showed no drastic difference in the endogenous expression levels of Grp94 and Grp78 mRNAs in mouse brain as well as neuro2a cells ( Fig. 6d ). These data support the specific reduction of Grp94 but not Grp78 by NF-Y suppression in brain neurons despite their similar expression in these tissues/cells. We further found specific accumulations of Ub, p62, APP or Calnexin in the cells with loss of Grp94 expression in NF-YA deletion mice, whereas KDEL was present in these cells ( Fig. 6e ). Quantitative analysis showed a gradual increase of Grp94-negative cells in which Ub and p62 exclusively accumulated ( Fig. 6f ). Thus, the loss of Grp94 expression induced by NF-Y suppression precedes accumulation of Ub and other proteins. Accumulation of misfolded proteins in ER is known to induce UPR, a major adaptive response to ER stress by activating several signalling cascades such as expressions of ER chaperons, CHOP and XBP1 (refs 26 , 27 , 28 ). No induction of ER chaperons by NF-Y suppression described above suggests the possibility that UPR is not induced despite abnormal accumulations of insoluble membrane proteins in ER of NF-YA deletion neurons. To confirm this, we checked UPR-related gene expressions and found no induction of CHOP/XBP1 expression or XBP1 splicing in NF-YA deletion mouse brain ( Fig. 7a,b ). Similarly, these are not induced in NF-YA/YC knockdown neuro2a cells ( Fig. 7c,d ). Finally, NF-YA/YC knockdown did not modulate ER stress-induced expressions of Grp78 and CHOP in neuro2a cells, whereas it suppressed basal and induced expressions of Grp94 ( Fig. 7e ). Taken together, these data suggest that NF-Y suppression does not induce or modulate UPR in neuronal cells but specifically affects Grp94 expression through direct regulation. 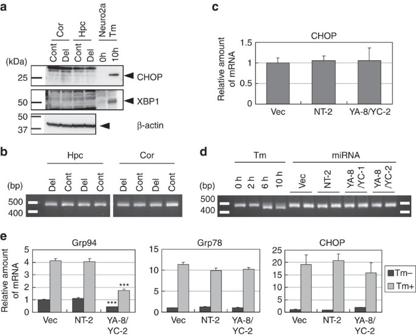Figure 7: Suppression of NF-Y does not cause distinct induction or modulation of UPR-related gene expression. (a) Isolated brain cortex (Cor) and hippocampus (Hpc) from 8-week-oldNF-YAflox/−; cre (Del) or flox/+ (Cont) mice were lysed and subjected to western blotting using antibodies for CHOP, XBP1 and β-actin. Lysates of neuro2a cells treated with 2.5 μg ml−1Tm for indicated hours were used as positive control. No distinct band for CHOP and XBP1 was observed in tissue lysates ofNF-YAdeletion mouse. Full-size blots can be found inSupplementary Fig. 15(b) RT–PCR for XBP1 splicing using isolated brain cortex (Cor) and hippocampus (Hpc) from 5-week-oldNF-YAflox/−; cre (Del) or flox/+ (Cont) female mice. No clear splicing (lower band) was observed in deleted mouse tissues. (c) Neuro2a cells were transfected with pcDNA6.2-EmGFP vector encoding tandem miRNAs for NF-YA and NF-YC (YA-8/YC-2), control miRNA (NT-2) or empty vector (Vec). After 3 days, the cells were subjected to quantitative RT–PCR to analyse CHOP expression. Values are means±s.d. of three experiments. (d) Transfected cells as in (c) or cells treated with 2.5 μg ml−1tunicamycin (Tm) for indicated hours were subjected to RT–PCR to monitor XBP1 splicing. Lower bands corresponding to spliced XBP1 were observed by Tm-treatment but not by NF-YA/NF-YC knockdown. (e) Transfected cells as in (c) were treated with or without 2.5 μg ml−1Tm for 10 h, and subjected to quantitative RT–PCR. Values are means±s.d. of three experiments (***P<0.001,t-test). Full-size gels can be found inSupplementary Fig. 14. Figure 7: Suppression of NF-Y does not cause distinct induction or modulation of UPR-related gene expression. ( a ) Isolated brain cortex (Cor) and hippocampus (Hpc) from 8-week-old NF-YA flox/−; cre (Del) or flox/+ (Cont) mice were lysed and subjected to western blotting using antibodies for CHOP, XBP1 and β-actin. Lysates of neuro2a cells treated with 2.5 μg ml −1 Tm for indicated hours were used as positive control. No distinct band for CHOP and XBP1 was observed in tissue lysates of NF-YA deletion mouse. Full-size blots can be found in Supplementary Fig. 15 ( b ) RT–PCR for XBP1 splicing using isolated brain cortex (Cor) and hippocampus (Hpc) from 5-week-old NF-YA flox/−; cre (Del) or flox/+ (Cont) female mice. No clear splicing (lower band) was observed in deleted mouse tissues. ( c ) Neuro2a cells were transfected with pcDNA6.2-EmGFP vector encoding tandem miRNAs for NF-YA and NF-YC (YA-8/YC-2), control miRNA (NT-2) or empty vector (Vec). After 3 days, the cells were subjected to quantitative RT–PCR to analyse CHOP expression. Values are means±s.d. of three experiments. ( d ) Transfected cells as in ( c ) or cells treated with 2.5 μg ml −1 tunicamycin (Tm) for indicated hours were subjected to RT–PCR to monitor XBP1 splicing. Lower bands corresponding to spliced XBP1 were observed by Tm-treatment but not by NF-YA/NF-YC knockdown. ( e ) Transfected cells as in ( c ) were treated with or without 2.5 μg ml −1 Tm for 10 h, and subjected to quantitative RT–PCR. Values are means±s.d. of three experiments (*** P <0.001, t -test). Full-size gels can be found in Supplementary Fig. 14 . Full size image Grp94 knockdown affects ER protein location in neuro2a cell The specific reduction of Grp94 without inducing UPR led us to hypothesize that NF-Y regulates ER organization through unidentified molecular mechanism. To examine this idea, we checked the effects of Grp94 knockdown on ER. We first confirmed specific downregulation of Grp94 by expressing our knockdown constructs, Grp94-1 and -5 ( Fig. 8e , Supplementary Fig. 11 ). Interestingly, Grp94 knockdown induced abnormal accumulation of ER luminal markers KDEL and PDI to the perinucler region in neuro2a cells ( Fig. 8a,b ). Significant local accumulations of these proteins were confirmed by quantitative analysis ( Fig. 8c ). In addition, the ER membrane protein Derlin1 also showed perinucler accumulation ( Fig. 8d ). In contrast, Grp78 knockdown (Grp78-2 and -10) did not change the localizations of KDEL or PDI, although it slightly reduced KDEL staining ( Fig. 8a,c,e ). Western blot analysis revealed no increase of KDEL or PDI by Grp94 knockdown ( Fig. 8e ), suggesting that the effect is not simply due to their induced expression. Importantly, Grp94 knockdown did not induce expression of CHOP or XBP1, which makes a clear contrast to the effect of Grp78 knockdown ( Fig. 8e ). Taken together, these data suggest that Grp94 knockdown induces abnormal local accumulation of ER without inducing UPR in neuro2a cells. No involvement of typical UPR pathways was confirmed by knocking down of ER stress-sensor proteins, that is, siRNA-mediated knockdown of Atf6, Perk or Ire1, which partly suppressed ER stress-induced UPR ( Supplementary Fig. 12 ), did not affect the local accumulation of KDEL and PDI induced by Grp94 knockdown ( Fig. 8f,g ). Using the neuro2a cellular system, we also found that knockdown of some of the other NF-Y target genes such as Hrd1 slightly induced local KDEL/PDI accumulation without significant induction of UPR ( Supplementary Fig. S13 ). Taken together, these data suggest that NF-Y may modulate ER organization through differential regulation of ER-related genes including Grp94 in neuronal cells. 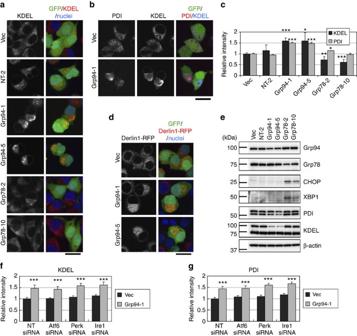Figure 8: Knockdown of Grp94 induces abnormal perinuclear accumulation of ER markers in neuro2a cells. (a,b) Neuro2a cells were transfected with pcDNA6.2-EmGFP vector encoding miRNA for Grp94 (Grp94-1 or -5), miRNA for Grp78 (Grp78-2 or -10), control miRNA (NT-2) or empty vector (Vec). After 2 days, cells were fixed and stained with anti-KDEL (a) or anti-PDI (b) together with DAPI. Confocal images are shown. (c) The intensities for KDEL and PDI in the GFP-positive cells (>600 cells per well) were quantified by Array Scan. Ratios to control (Vec) are shown. Values are means±s.d. of six (KDEL) or three (PDI) experiments (*P<0.05, **P<0.01, ***P<0.001,t-test). (d) Neuro2a cells stably expressing Darlin1-RFP were transfected with pcDNA6.2-EmGFP vector encoding miRNA for Grp94 (Grp94-1 or -5) or empty vector (Vec). After two days, cells were fixed and analysed by confocal microscope. (e) Neuro2a cells transfected with pcDNA6.2-EmGFP vector encoding indicated miRNAs or empty vector for 2 days were subjected to western blotting with antibodies for indicated proteins. Full-size blots can be found inSupplementary Fig. 15. (f,g) Neuro2a cells were first transfected with siRNA for Atf6, Perk, Ire1 or non-targeting control (NT) for 1 day. Then, the cells were transfected with pcDNA6.2-EmGFP vector encoding Grp94-1 miRNA or empty vector (Vec). After 2 days, cells were fixed and stained as in (b). KDEL (f) or PDI (g) fluorescence intensities were analysed as in (c). Values are means±s.d. of six experiments (***P<0.001,t-test). Scale bars are 20 μm (a,b,d). Figure 8: Knockdown of Grp94 induces abnormal perinuclear accumulation of ER markers in neuro2a cells. ( a , b ) Neuro2a cells were transfected with pcDNA6.2-EmGFP vector encoding miRNA for Grp94 (Grp94-1 or -5), miRNA for Grp78 (Grp78-2 or -10), control miRNA (NT-2) or empty vector (Vec). After 2 days, cells were fixed and stained with anti-KDEL ( a ) or anti-PDI ( b ) together with DAPI. Confocal images are shown. ( c ) The intensities for KDEL and PDI in the GFP-positive cells (>600 cells per well) were quantified by Array Scan. Ratios to control (Vec) are shown. Values are means±s.d. of six (KDEL) or three (PDI) experiments (* P <0.05, ** P <0.01, *** P <0.001, t -test). ( d ) Neuro2a cells stably expressing Darlin1-RFP were transfected with pcDNA6.2-EmGFP vector encoding miRNA for Grp94 (Grp94-1 or -5) or empty vector (Vec). After two days, cells were fixed and analysed by confocal microscope. ( e ) Neuro2a cells transfected with pcDNA6.2-EmGFP vector encoding indicated miRNAs or empty vector for 2 days were subjected to western blotting with antibodies for indicated proteins. Full-size blots can be found in Supplementary Fig. 15 . ( f , g ) Neuro2a cells were first transfected with siRNA for Atf6, Perk, Ire1 or non-targeting control (NT) for 1 day. Then, the cells were transfected with pcDNA6.2-EmGFP vector encoding Grp94-1 miRNA or empty vector (Vec). After 2 days, cells were fixed and stained as in ( b ). KDEL ( f ) or PDI ( g ) fluorescence intensities were analysed as in ( c ). Values are means±s.d. of six experiments (*** P <0.001, t -test). Scale bars are 20 μm ( a , b , d ). Full size image Using gene deletion or knockdown strategies, we here showed that suppression of NF-Y in brain differentiated neurons resulted in progressive neurodegeneration accompanying insolubilization of Ub and p62 and their accumulation on ER. It also induced accumulation of insoluble integral membrane proteins on ER and drastic increase in SER in degenerating neurons. We further identified several NF-Y target genes including Grp94 by ChIP–chip, and found that knockdown of some of them induced abnormal perinuclear accumulation of ER markers in neuro2a cells. These data indicate that NF-Y is involved in the regulation of ER organization in neuronal cells and its disruption results in cell loss with atypical neurodegenerative features including Ub/p62 accumulation on ER and abnormal SER increase. Ub, an essential mediator of protein degradation through proteasomes, is known to be accumulated in inclusions containing fibrillar protein aggregates in various neurodegenerative diseases [20] . p62, a key regulator for selective degradation of ubiquitinated proteins through autophagy, is also often found in the inclusions [21] . Although Ub and p62 were insolubilized in NF-YA deletion mice brains, they were broadly located on the ER ( Figs 3 and 4 ). In addition, western blot and mass spectrometry analyses indicated no insolubilization of known aggregation-prone proteins in these mice brains ( Supplementary Fig. 6 , Supplementary Table 2 ). Furthermore, EM and immuno-EM analyses revealed no obvious filamentous structures around the ER in degenerating neurons ( Fig. 4 ). These data suggest that Ub and p62 are not contained in the inclusion with fibrillar protein aggregates, but entirely localized to ER together with insolubilized membrane proteins. Thus, the Ub/p62 pathology observed here is very specific to the NF-YA deletion neurons and different from the general pathologies observed in many neurodegenerative diseases. Although target proteins of Ub and p62 for degradation have not been identified in this study, co-accumulation of integral membrane proteins implies that some of them are the potential substrates. Thus, one simple explanation of Ub/p62 accumulations would be overload of insoluble membrane proteins, which affects their efficient degradation through the proteasome and autophagy systems. Alternatively, potential cytoplasmic compartmentalization induced by increased SER could lead to local deficiency in cytoplasmic components involved in these degradation systems. Indeed, we found that accumulated p62 was phosphorylated at its S403 residue and colocalized with LC3 ( Supplementary Fig. 3a,b ), a potential intermediates of p62-mediated autophagy [29] . In addition, western blot analysis showed the accumulation of LC3-II in addition to phosphorylated p62 ( Supplementary Fig. 5a,b ). These data imply impairment of autophagy flux in NF-YA deletion neurons. As p62 accumulation was specifically observed around the abnormal ER ( Figs 3e and 4h ), whereas distinct accumulation of autophagosomes was not observed by our EM analysis, it is possible that ER-specific autophagy such as reticulophagy is impaired at the very early stage of the flux. In addition, a subtle reduction of proteasome activity was observed in cortical lysates of NF-YA deletion mice ( Supplementary Fig. 3c,d ). Although further analysis is necessary for full understanding of atypical accumulation of Ub and p62, perturbation of the degradation systems around ER could be involved in some aspects of neurodegeneration in NF-YA deletion mice. Despite the abnormal accumulations of insoluble proteins on ER, the degeneration did not accompany an ER stress response (UPR) ( Fig. 7 ), but a drastic increase in SER ( Fig. 4 ) in NF-YA deletion mice brains. Although the mechanism of SER increase without UPR remains obscure, several in vitro studies have shown that ectopic expression of a single ER-resident membrane protein, such as cytochrome b(5) and calnexin, induces SER proliferation [30] , [31] , [32] , [33] , [34] . In addition, this phenomenon does not involve typical UPR nor requires the ER stress sensors, and thus is suggested to be another adaptive response of ER for overload of membrane proteins [31] , [35] , [36] . As insolubilization was so far selective for membrane proteins in NF-YA deletion mice brains ( Fig. 3 ), it is possible that this selective insolubilization may mediate the SER proliferation without causing UPR in NF-YA deletion neurons. Notably, the accumulation in ER and associated SER proliferation is also observed in cultured cells by ectopic expression of mutant VAMP-associated protein B (VAPB), a causative protein of amyotrophic lateral sclerosis-8 (refs 37 , 38 ). Thus, it would be worthwhile to analyse human patient tissue with the disease mutation, which may lead to establish a novel, ER stress-independent human neuropathology as observed in our mutant mice. So, how does NF-Y suppression mediate ER disorganization? We here found that NF-Y suppression selectively downregulated Grp94 but not Grp78 in vitro and in vivo ( Fig. 6 ). In addition, knockdown of Grp94 but not Grp78 induced distinct perinuclear accumulation of several ER markers in neuro2a cells independently of ER stress sensors ( Fig. 8 ). Finally, Grp94 knockdown did not involve UPR, whereas Grp78 knockdown induced it ( Fig. 8 ). These observations suggest that selective downregulation of Grp94 seems to be a key event of ER disorganization without inducing UPR. The differential regulation of Grp94 and Grp78 by NF-Y may not be due to the difference in the basal expression level because their expression level is relatively similar in mouse brain and neuro2a cells ( Fig. 6d ). In contrast to the cells analysed here, NF-Y suppression is shown to induce Grp78 downregulation in some cultured cell lines [25] , [39] , and NF-YA deletion in mouse hepatocytes is reported to induce Grp78 expression and UPR followed by cell degeneration [40] . Thus, the molecular basis of dysregulation of ER chaperones and ER pathologies by NF-Y suppression is different among cell types, and neuron-specific dysregulation would be the cause of unique degenerative features observed in NF-YA deletion mice. Although the mechanism of ER mislocalization by Grp94 knockdown is unclear, no effect by Grp78 knockdown supports the idea that it may not be due to global impairment of protein folding in ER, rather due to the suppression of Grp94-specific function. This could include folding of Grp94-specific client proteins, whose disruption results in their misfolding and accumulation in ER, leading to ER morphological alteration. Alternatively, Grp94 itself could have a direct role in ER organization. Despite the local accumulation of ER luminal and membrane proteins, their protein levels were not increased by Grp94 knockdown in neuro2a cells ( Fig. 8 ), implying that Grp94 knockdown just alters ER location/organization but does not induce drastic ER disorganization such as ER proliferation/expansion as observed in NF-YA deletion mice neurons. Notably, we found that AAV-mediated knockdown of Grp94 in mouse brain did not induce obvious neuronal loss or Ub accumulation ( Supplementary Fig. 11a ). These data support the notion of insufficiency of only Grp94 downregulation for neurodegeneration and suggest requirement of co-suppression of other NF-Y targets to reproduce the pathologies caused by NF-Y inactivation in vivo . We also noticed that Grp78 was significantly increased in Grp94 knockdown cells ( Supplementary Fig. 11b–d ), implying potential compensation of the loss of Grp94 by increased Grp78 in the presence of NF-Y in brain neurons. Further analysis is necessary for full understanding of the pathomechanism of neurodegeneration induced by NF-Y inactivation. Previously, we found that NF-YA is incorporated into nuclear inclusion in HD model mice brains, leading to suppression of NF-Y mediated gene expression [13] . Although atypical Ub/p62 accumulation as observed in NF-YA deletion mice is not observed in HD, ER abnormalities such as ER cisternal extension and ribosomal depletion are observed in HD patient brain neurons [41] . In addition, nuclear indentation is reported in brain neurons of HD model mice [42] . Thus, some of the mechanisms identified here might also be involved in some aspects of HD pathogenesis. In summary, we found that NF-Y suppression in differentiated mouse brain neurons induced novel neuropathology with distinctive Ub/p62 accumulation, which was completely different from the pathology induced by ER stress. We propose that NF-Y modulates ER organization possibly through neuron-specific mechanism involving selective regulation of ER chaperones. Further analysis may provide novel aspects of neuropathology involving Ub/p62 accumulation. Mice The mouse experiments were approved by the animal experiment committee at RIKEN Brain Science Institute. Mice were maintained and bred in accordance with RIKEN guidelines. NF-YA flox mice ( Fig. 1a ) [2] were maintained on a C57BL6 (B6) background by mating with female B6 mice. The camk2a-cre transgenic mice harbouring a transgene containing cre recombinase under the camk2a promoter [16] were obtained from the Jackson Laboratory (Bar Harbor, ME). CAG-cre transgenic mice [43] and RNZ ( ROSA26-loxP-STOP-loxP-nlsLacZ ) mice [18] were generously provided by Dr Miyazaki (Osaka University) and Dr Itohara (RIKEN BSI), respectively. All mice were maintained on a B6 background. The cre;RNZ mice were generated by crossing camk2a-cre mice with RNZ mice. For generation of RNZ mice harbouring NF-YA flox/−; cre, NF-YA +/− cre; RNZ mice were first generated and crossed with NF-YA flox/flox mice. The NF-YA heterozygous mice (+/−) were generated by crossing NF-YA flox/+ mice with CAG-cre transgenic mice. The sequences of primers used for genotyping are described in Supplementary Table 3 . We mainly used male mice for most of the analyses except of indication of usage of female mice for analysis. Age of the mice used for analyses are described in the figures or figure legends. Generation of NF-YA conditional deletion mice We first tried the usual strategy to generate neuron-specific NF-YA conditional deletion mice by crossing NF-YA flox/+; cre mice with NF-YA flox/flox mice ( Supplementary Table 4 ). However, mice harbouring NF-YA flox/flox; cre were hardly obtained, probably due to a strong linkage between NF-YA wild-type (+) locus and cre locus and thus very low frequency of homologous recombination between these loci. Accidentally, we did obtain one mouse harbouring NF-YA flox/+; cre showing strong linkage between NF-YA flox locus and cre locus, that is, when crossed with flox/flox mouse, most of the resultant pups harboured flox/+ or flox/flox; cre ( Supplementary Table 5 ). Unexpectedly, some flox/−; cre mice were also obtained possibly because of instability of one of NF-YA flox alleles in the presence of camk2a-cre transgene in germ line. We also obtained an NF-YA +/−; cre mouse in which the deleted allele (−) and cre loci were strongly linked. As expected, when crossed with flox/flox mice, most pups harboured flox/−; cre or flox/+ at a nearly 1:1 ratio ( Supplementary Table 6 ). Antibodies Polyclonal antibodies for NF-YA (YA-2-3, 1:500 dilution), NF-YC (YC6-3, 1:200), TLS (TLS-M, 1:1,000) and α-synuclein (S1, 1:500) were generated in rabbit [13] , [44] , [45] , and a monoclonal antibody for phospho-S403 of p62 (4F6, 1:500) was generated in rat [29] . Antibody for USF1 (C-2, 1:300) was generated in rabbit against the C-terminal 15 a.a. of mouse USF1 and purified by antigen peptide conjugated to SulfoLink Coupling Gel (PIERCE). Antibodies for CPE (610758, 1:1,000), GM130 (610822, 1:500), Grp78 (610978, 1:2,000), Rab3 (610379, 1:500), Tau (T57120, 1:500) and Rab11 (R56320, 1:500) were from BD (Transduction); GFAP (Z0334, 1:2,000) and Ub (Z0458, 1:500) from DAKO; CHOP (ALX-804-551, 1:2,000), Calnexin (SPA-860, 1:500), Grp94 (SPA-850, 1:2,000), PDI (SPA-891, 1:2,000) and ubiquitin (FK2, BML-PW8810, 1:1,000) from Enzo; GFP (598, 1:1,000), KDEL (PM059, 1:2,000), p62 (PM045, 1:1,000) and LC3 (PM045, 1:500) from MBL; APP (MAB348, 1:1,000), Calnexin (AB1769, 1:500), NeuN (MAB377, 1:200) and Ub (MAB1510, 1:20,000) from MILLIPORE (Chemicon), HSP 60 (K-19) (sc-1722, 1:500), NF-YA (sc-10779, 1:100), USF1 (sc-229, 1:200), Enolase (sc-7455, 1:500), Rab6 (sc-310, 1:500) and XBP1 (sc-7160, 1:300) from Santa Cruz; β-actin (A5441, 1:1,000) from Sigma-Aldrich. The following antibodies were also used: Calreticulin (2891, Cell Signalling, 1:200), p62 (GP62-C, PROGEN, 1:2,000), TDP-43 (10782-2-AP, Proteintech, 1:1,000), GFP (1814460, Roche, 1:1,000), LacZ (200-4136, Rockland, 1:1,000), ARF (MA3-060, ABR, 1:500) and Iba1 (019-19741, WAKO, 1:500). Plasmids miRNA expression vectors for NF-YA (YA-8), NF-YC (YC-1, YC-2), Grp94 (Grp94-1, -5), Grp78 (Grp78-2, -10), other NF-Y target genes (Calnexin, Cnpy3, Dnajb5, Hrd1, Kdelc1, Rab5b, Sdf2l1, Sec61g, Tpcn1, Usp5 and Yif1a) and control non-targeting miRNA (NT-2) were generated using the pcDNA6.2-GW/EmGFP-miR vector (Invitrogen). In this system, miRNA expression could be monitored by EmGFP expression. The oligonucleotide sequences used for construction are listed in Supplementary Table 7 . Tandem miRNAs expression vector containing two miRNAs (YA-8/YC-2 or Grp94-1/-5) were generated by insertion of one of miRNA into another according to the manufacturer’s protocol. Mouse cDNAs for Grp94 and Grp78 were kindly provided as FANTOM [46] and subcloned into pcDNA3.1 vector, which were used to compare the respective endogenous levels of these two genes by quantitative PCR. Histological analysis Mice were perfused with 4% paraformaldehyde (PFA)/phosphate-buffered saline (PBS). Isolated brains were further fixed overnight with 4% PFA/PBS, cryoprotected with 20% sucrose/PBS, frozen in tissue mount and processed for cryosectioning (10 μm). Hematoxylin staining was performed using Mayer’s Hematoxylin. For immunohistochemistry and immunofluorescence analysis [47] , cryosections were autoclaved in 10 mM citrate buffer (pH 6.0) at 120 °C for 5 min, treated with 0.01% H 2 O 2 /methanol at room temperature for 30 min and blocked with 5% skim milk/TBST (20 mM Tris–HCl, pH 8.0, 150 mM NaCl, 0.05% Tween20) for 1 h. The sections were then incubated with a primary antibody diluted with TBST containing 0.1% bovine serum albumin (BSA) for overnight at 4 °C. For immunohistochemistry, they were then incubated with a secondary antibody conjugated with horseradish peroxidase (Vector), and then with ABC regent (Vector), followed by detection with diaminobenzidine (DAB). For immunofluorescence, the sections were incubated with a secondary antibody conjugated with Alexa Fluor dyes (Molecular Probes). Images were obtained on a CCD camera-equipped Olympus microscope (AX80), Keyence microscope (BZ-9000) or Leica confocal system (TCS SP2). RT–PCR and gene expression microarray For brain tissues, total RNA was prepared using Trizol (Invitrogen) and RNeasy kit (Qiagen) according to the manufacturers’ protocols. For neuro2a cells, total RNA was directly prepared using RNeasy kit. These RNAs were subjected reverse transcription using ThermoScript RT–PCR Systems (Invitrogen) to synthesize cDNA according the manufacturer’s protocol. Primers and TaqMan probes for quantitative PCR listed in Supplementary Table 8 were designed based on Primer Express software (Applied Biosystems). Quantitative PCR was performed by TaqMan or SYBR green according to the manufacturer’s protocol (Applied Biosystems or Roche). All values obtained were normalized with respect to levels of GAPDH mRNA. XBP1 splicing was detected by PCR amplification of its splicing site from cDNAs using the following primers, 5′-AAACAGAGTAGCAGCGCAGACTGC-3′ and 5′-TCCTTCTGGGTAGACCTCTGGGAG-3′ (ref. 48 ). Full-size images of gel electrophoresis are presented in Supplementary Fig. 14 . For gene expression microarray, labelled cDNA probes were prepared from total RNA by Ambion WT Expression Kit and Affymetrix WT Terminal Labeling Kit according to the manufacturer’s protocol. The probes were hybridized to Affymetrix Mouse Gene ST array and the obtained data were analysed using Agilent GeneSpring GX 10 software. Stereotaxic injection of AAV vectors for miRNAs The AAV vectors expressing EmGFP with tandem miRNA (YA-8/YC-2 or Grp94-1/5) or control miRNA (NT-2) under CAG promoter were prepared by GeneDetect. To inject AAV into brain hippocampus, 6-week-old wild-type male B6 mice were first anaesthetized by peritoneal injection of pentobarbital and placed in a stereotaxic apparatus. A total of 3 × 10 9 genomic particles of AAVs were injected through burr holes in the skull. Injection was placed at 2.5 mm posterior to the bregma, 2 mm lateral to the sagittal suture and 1–1.5 mm below the skull surface. Brain fractionation and western blot Isolated brain cortexes were suspended in RIPA buffer containing 20 mM Hepes at pH 7.2, 150 mM NaCl, 1 mM EDTA, 1 × Complete, 1% triton X-100, 0.5% deoxycholate and 0.1% SDS with teflon homogenizer on ice. After sonication and quantification of protein concentration, 150 μl homogenates containing 1 mg protein were subjected to ultracentrifugation at 50,000 r.p.m. for 30 min at 4 °C with TLA-55 rotor (Beckman). The supernatants (S1) were removed and pellets were briefly sonicated in 150 μl of 1% sarcosyl in RIPA buffer and centrifuged as above. After removal of the supernatants (S2), the pellets were further solubilized with 4% sarcosyl in RIPA buffer (S3) as above. Remaining pellets (P) were then solubilized with 100 μl of formic acid at 37 °C for 1 h and dried by vacuum centrifugation. After boiling in SDS sample buffer, these fractions (S1–S3 and P) were subjected to SDS-PAGE and blotted on PVDF membrane. After blocking with 5% skim milk/TBST, the membrane was incubated with a primary antibody diluted in TBST containing 5% goat serum and then with a secondary antibody conjugated with horseradish peroxydase in same buffer [49] . Chemiluminescent signals were obtained and quantified using ImageQuant LAS-4000 (GE). Full-size images of western blot are presented in Supplementary Fig. 15 . Mass spectrometry For identification of insoluble proteins, the 4% sarcosyl-insoluble (P) fractions from 14-week-old NF-YA flox/−; cre and flox/+ female mice cortexes were separated by SDS-PAGE, stained briefly with SymplyBlue SafeStain (Invitrogen), and cut into 10 pieces ( Supplementary Fig. 6b ). The gels were then treated with 10 mM dithiothreitol/100 mM NH 4 HCO 3 at 50 °C for 15 min, and with 10 mM iodoacetamide/100 mM NH 4 HCO 3 at room temperature for 15 min, followed by incubation with 10 μg ml −1 trypsin at 37 °C for overnight. After extraction with 1% trifluoroacetic acid/50% CH 3 CN, obtained peptides were first separated by a Paradigm MS2 HPLC system (Michrom BioResources), ionized with a Nanoflow-LC ESI, and then analysed using an LTQ linear ion trap mass spectrometer (Thermo Fisher Scientific) to obtain MS/MS spectrum data of the peptides. Based on this peptide information, proteins were identified using Mascot software (Matrix Science). Proteasome activity assay Isolated brain cortexes were suspended in lysis buffer containing 50 mM Tris–HCl at pH 7.5, 250 mM sucrose, 25 mM KCl, 10 mM NaCl, 1 mM MgCl 2 , 1 mM ATP and 10% glycerol with teflon homogenizer on ice. After sonication and centrifugation at 20,000 g for 30 min at 4 °C, protein concentration was measured by Bradford method. The lysates containing 25 μg protein were mixed with 100 μM Suc-LLVY-AMC (Enzo) in assay buffer containing 50 mM Tris–HCl at pH 7.5, 25 mM KCl, 10 mM NaCl, 1 mM MgCl 2 and 1 mM ATP, and chymotryptic-like activity was examined by measuring free AMC fluorescence using a Perkinelmer EnVision plate reader. EM and immuno-EM For conventional EM, mice were perfused with 0.1 M phosphate buffer (PB) (pH 7.4) containing 2% PFA and 2.5% glutaraldehyde. Brains were sectioned at 500 μm, osmicated with 1% OsO 4 in phosphate buffer, dehydrated through a gradient series of ethanol and then embedded in epoxy resin (Epon 812, TAAB). Ultrathin sections (80 nm thick) were made with an ultramicrotome (Ultracut UCT or UC6, Leica) and collected on 200-mesh uncoated copper grids. After counterstaining with uranyl acetate and lead citrate, the sections were examined with FEI Tecnai 12 or Hitachi HT7700 electron microscopy. For immuno-EM using ultrathin cryosections [50] , [51] , mice were perfused with 4% PFA/PBS and isolated brains were immersed in the same buffer for 3 h. The hippocampal CA1 region was cut into small pieces, washed thoroughly with 7.5% sucrose/PB, embedded in 12% gelatin and rotated in 2.3 M sucrose/PB overnight at 4 °C. Ultrathin cryosections ~60 nm thick were prepared with Leica UC7/FC7. The sections were rinsed with PBS containing 0.02 M glycine, treated with 1% BSA in PBS and incubated overnight at 4˚C with rabbit anti-p62 (PM045) (1:10) and mouse anti-ubiquitin (FK2) (1:10). The sections were then incubated with anti-rabbit and anti-mouse IgG conjugated with 10 nm and 5 nm colloidal gold particles (1:40) (British Biocell International), respectively, for 1 h at room temperature, and examined with a Hitachi H-7100 electron microscope. Chromatin immunoprecipitation Frozen isolated brain cortexes were broken into small pieces using mortar and pestle and fixed with 10 v / w of 1% formalin/PBS at 37 °C for 10 min to crosslink the transcription factor (TF)-–DNA complex. After adding 0.1 v / v of 1 M glycine/PBS and brief centrifugation, the pellets were homogenized in 5 v / w of SDS lysis buffer (1% SDS, 10 mM EDTA, 50 mM Tris, pH 8.0, 1 × Complete) with teflon homogenizer for 30 strokes. The homogenates were sonicated for 20 s 5 times and centrifuged at 20,000 g for 10 min. The supernatants were diluted 10-fold with ChIP dilution buffer (0.01% SDS, 1.1% Triton X-100, 1.2 mM EDTA, 16.7 mM Tris–HCl, pH 8.0, 167 mM NaCl, 1 × Complete) and 1 ml aliquots (Inputs) were stored at −80 °C. ChIP was performed using the inputs according the ChIP Assay Kit protocol (Millipore). Note that salmon sperm DNA was excluded in case of ChIP–chip because it increases non-specific signals in the array. The ChIP samples were analysed by PCR or real-time PCR using primers listed in Supplementary Table 9 . Full-size data of gel electrophoresis are presented in Supplementary Fig. 14 . ChIP–chip For promoter array analysis (ChIP–chip), the ChIP DNAs were linear-amplified with sequenase, amplified with rTaq polymerase and then labelled with biotin according to the Affymetrix ChIP Assay Protocol. The labelled DNAs were hybridized to a Affymetrix GeneChip Mouse Promoter 1.0R Array, a single array comprising >4.6 million probes tiled to over 28,000 mouse promoter regions where approximately −6 kb to +2.5 kb of 5′ TSSs are covered. The obtained data were analysed using CisGenome software [23] to identify TF binding regions with significant fold changes by comparison of each of ChIP–chip data with that of control IgG. By using the software, we also annotated TF binding regions with their neighbour genes (±10,000 bp from TSSs). As only one gene could be identified by this procedure, we rechecked TF-binding regions manually to search for other genes located adjacent to the ones identified in the top 400 annotated regions detected by ChIP. We further identified the TF-binding consensus sequence and analysed its enrichments or positions from TSSs using this software. Cell culture and transfection Neuro2a mouse neuroblastome cells, a gift from Dr Iwatsubo (Tokyo University) [52] , were maintained in DMEM supplemented with 10% FBS and penicillin–streptomycin in an atmosphere containing 5% CO 2 . Transfection was performed by Lipofectamine 2000 (Invitrogen) according to the manufacturer’s protocol. To establish a neuro2a cell line stably expressing Derlin1-RFP, neuro2a cells were transfected with pmRFP-N1 vector containing mouse Derlin1 by Lipofectamine 2000 and incubated with culture media containing 300 μg ml −1 G418. For knockdown of ER stress-sensor proteins, siRNAs (ON-TARGETplus SMARTpool) for Atf6, Perk and Ire1 were purchased from Dharmacon, and introduced into cells using RNAiMAX (Invitrogen) according to the manufacturer’s protocol. For immunofluorescence analysis [53] , cells were fixed with 4% PFA/PBS, permeabilized with 0.1% triton X-100/TBST and blocked with 5% goat serum/TBST. The cells were then incubated with primary antibody diluted with 0.1% BSA/TBST and then with secondary antibody conjugated with Alexa Fluor dyes. Images were obtained by Leica confocal system (TCS SP2). Cell image analysis For quantitative analysis of fluorescence of neuro2a cells seeded on culture plate, we used the ArrayScan VTI HCS Reader (Cellomics, Thermo Fisher Scientific). Protocols were designed according to the instruction manual. Cell images were not obtained randomly, but those in same area of each well were automatically obtained using equipped fluorescence microscopy to equate the analyses among the wells. Then, intensities of KDEL or PDI regions in GFP-positive transfected cells were analysed. For quantitative analysis of fluorescence of mouse brain cortex, at least four fields containing almost same cortical area among different samples were obtained and analysed manually. For analysis of LacZ-positive cells in CA1 region, a field of each hemisphere was obtained and CA1 cell number in 100 μm in width was counted manually. GO analysis GO term enrichment analysis was performed by GO:TermFinder software [22] on the AmiGO website ( http://amigo.geneontology.org/cgi-bin/amigo/go.cgi ). Statistical significance was calculated by this software and P <0.05 was considered significant. Statistical analysis Sample sizes were chosen on the basis of pilot experiments and previous experience with similar types of experiments. For comparison between two sample groups, data were first analysed by F-test. For P <0.05, the data were analysed by unpaired Student’s t -test (two-tailed); otherwise, data were analysed by Welch’s t -test (two-tailed). For survival rate we plotted the survival distribution curve with the Kaplan–Meier method followed by log-rank testing (JMP Statistical Discovery software). We considered the difference between comparisons to be significant when P <0.05 for all statistical analyses. No data points were excluded in the analysis. All of the experiments were successfully repeated at least two times. How to cite this article: Yamanaka, T. et al. NF-Y inactivation causes atypical neurodegeneration characterized by ubiquitin and p62 accumulation and endoplasmic reticulum disorganization. Nat. Commun. 5:3354 doi: 10.1038/ncomms4354 (2014).